Metasurface holograms for visible light Holography, a revolutionary 3D imaging technique, has been developed for storing and recovering the amplitude and phase of light scattered by objects. Later, single-beam computer-generated phase holography was proposed for restoring the wavefront from a given incidence. However, because the phase modulation depends on the light propagation inside the material, the thickness of phase holograms usually remains comparable to the wavelength. Here we experimentally demonstrate ultra-thin metasurface holograms that operate in the visible range whose thickness is only 30 nm (approximately 1/23 of the operational wavelength). To our knowledge, this is the thinnest hologram that can provide both amplitude and phase modulation in the visible wavelength range, which generates high-resolution low-noise images. Using this technique, not only the phase, but potentially the amplitude of the incident wave can be efficiently controlled, expanding the route to new applications of ultra-thin and surface-confined photonic devices. Traditional two-beam holography relies on recording the interference pattern of the scattered light and a coherent reference beam [1] , [2] . This technique produces an amplitude hologram through which the scattered wavefront is directly recorded through the intensity of the interference pattern. By translating the intensity variations in the interference pattern into phase variations, one may build a phase hologram, which increases the brightness of the image substantially [3] , [4] . In contrast to two-beam holography, one of the earliest computer-generated phase holograms, a kinoform [5] , [6] , has been designed as a complex lens which transforms a given incident wavefront into the transmitted wavefront used to recreate the desired image. To restore the image, this phase hologram uses a single diffraction order, which (in the ideal case) includes all of the spatial modes of the modulated incident light. This hologram has utilized only the phase of an incident wave, whereas the amplitude of the wavefront in the hologram plane has been assumed constant [5] , [6] . The progression of micro- and nano-scale lithographic fabrication has revitalized the area of computer-synthesized phase holograms through controlling the phase with pixelated arrays of structural unit cells made of single-layer subwavelength-pitch dielectric gratings [7] , dielectric optical antennas [8] or multilayer metamaterial media [9] , [10] . The computer-generated approach to designing these phase holograms has already resulted in sophisticated applications [11] , which are extremely difficult to obtain with a fully optical recording process. Because the phase modulation in the above phase holograms relies on dielectric optical antennas or the difference of the refractive index changes in a transparent layer, the complete phase control requires the wavelength-scale or even larger size of unit cells and/or thickness of the phase hologram. Optical metasurfaces, the basis for our computer-synthesized and nano-fabricated hologram, have already exhibited unusual phenomena in ways that traditional optical materials, coatings and devices are unable to duplicate [12] , [13] , [14] , [15] , [16] , [17] , [18] , [19] , [20] , [21] , [22] , [23] , [24] . The field of metasurfaces is rapidly expanding, and have already been used to bend light abnormally [12] , [19] , rotate polarization [25] , engineer the optical spin–orbital interaction [23] , [24] , create [12] , [15] or detect [20] optical vortex beams, couple propagating waves to surface waves [17] , and create ultra-thin planar lenses [18] , [26] , [27] , [28] , [29] . In this article, we experimentally demonstrate an advanced hologram (compare, for example, refs 30 , 31 ) recorded as a nanostructured plasmonic metasurface [32] , which directly records both the amplitude and phase of the wavefront scattered by an object. Similar to the kinoform, our approach requires no reference beam and generates no conjugate image, as all the spatial bandwidth of the metasurface hologram is utilized in a holographic picture. Furthermore, as the metasurface hologram modulates both amplitude and phase on a subwavelength scale, the proposed approach can achieve conceptually much higher diffraction efficiency (the fraction of the transmitted energy of the cross-polarized light that contributes into the holographic image) than traditional holograms as all the orders of diffraction fully contribute to the holographic image. At the same time ultra-thin, ultra-small holograms can now be recorded, providing unprecedented spatial resolution, low noise, and high precision of the reconstructed image. Conventionally, a phase hologram is made by engineering the local optical path by changing either the thickness or the refractive index of a material layer [33] , [34] . In ref. 9 a multilayer, graded-index metamaterial has been used to demonstrate a mid-infrared phase hologram, where the required phase modulation was provided by local optical paths through a structure with a thickness on the order of the incident wavelength. In this study, we demonstrate holographic images generated at a wavelength of 676 nm by a 30-nm thick planar metasurface hologram, consisting of an array of phase-controlling plasmonic nanoantennas. Metasurface hologram design principles To create the metasurface hologram, we use a set of the Babinet-inverted, complementary nanoantennas (CNAs)—nano-voids of different shapes perforated in a thin, metallic film on a glass substrate. Each CNA shape provides a specific phase shift to the cross-polarized, scattered light (that is, the scattered polarization is perpendicular to the incident polarization, see Methods section). As the CNAs scatter both co-polarized and cross-polarized light, we cannot totally eliminate the co-polarized component. However, the complementary design efficiently prevents the direct transmission of the co-polarized component as the rest of the sample remains opaque owing to the continuous metallic film. To design the metasurface hologram, we first choose an image plane and selected a virtual object to be generated in that plane. We have taken the word ‘PURDUE’ as our test virtual object. Next, we consider the test object to emit 676-nm linearly polarized coherent light, and we mapped the phase and amplitude of the electric field onto the metasurface hologram plane (which was taken 10 μm below and parallel to the image plane). A more detailed explanation of the constructing procedure can be found in the Methods section. 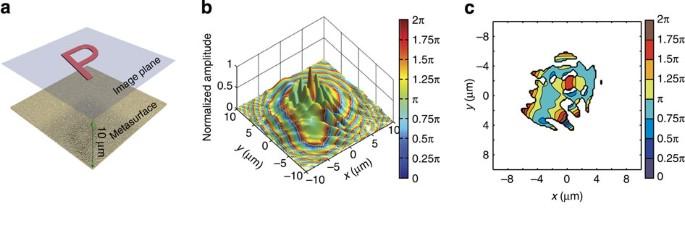Figure 1: Metasurface hologram design steps. (a) An image plane is chosen above the metasurface hologram at a given distance (here we choose 10 μm). A flat, light-emitting virtual object is located in the image plane. The phase and amplitude distribution of the electric field propagating from the object are mapped to the metasurface plane. (b) The calculated amplitude (zvalue) and phase distribution (pseudo-colour map) on the metasurface plane. (c) The discrete eight-level phase distribution with a two-level amplitude modulation to accommodate the antenna designs. The blank areas indicate the ‘off’ state and also correspond to ‘blank’ pixels. Figure 1a illustrates this design step by using the first letter ‘P’ of the virtual object. The metasurface hologram area is then covered with a uniform grid of square cells (pixels). A subwavelength-sized (150 × 150 nm 2 ) pixel is sufficiently large to accommodate an individual antenna and to prevent cross-talk between adjacent pixels. The phase modulation is accomplished by approximating the phase map with eight discrete phase levels, which are then reproduced by eight distinct antenna shapes inside each pixel. The calculated amplitude and phase distribution for the letter ‘P’ is shown in Fig. 1b . Although it is possible to control both the phase and amplitude of the cross-polarized light by changing the design parameters of the CNAs (see Methods section, in which we give the design parameters for an eight-level phase and four-level amplitude modulation), for simplicity we use a fixed, average amplitude in our design. Hence, the amplitude modulation is achieved by just two states (on and off) with a chosen threshold (that is, by introducing a pixel either with or without an antenna). Figure 1c shows the simplified discrete phase map using this two-level amplitude modulation. The blank areas indicate pixels without antennas. Note that the rapid phase-change areas in the off-centre region of Fig. 1b are pixels with very small amplitudes. Those areas are all in the ‘off’ state, and therefore have no antennas. Figure 1: Metasurface hologram design steps. ( a ) An image plane is chosen above the metasurface hologram at a given distance (here we choose 10 μm). A flat, light-emitting virtual object is located in the image plane. The phase and amplitude distribution of the electric field propagating from the object are mapped to the metasurface plane. ( b ) The calculated amplitude ( z value) and phase distribution (pseudo-colour map) on the metasurface plane. ( c ) The discrete eight-level phase distribution with a two-level amplitude modulation to accommodate the antenna designs. The blank areas indicate the ‘off’ state and also correspond to ‘blank’ pixels. Full size image The holographic image is simulated by substituting each CNA with a point source of cross-polarized light with a corresponding phase. The overall light intensity profile of a given hologram is then calculated as the superposition of the field from the entire grid of point sources. For our experiments, the initial 30-nm-thick continuous gold film was deposited on a glass substrate with electron-beam vapour deposition. The samples were then milled to their desired shape using a focused ion beam. 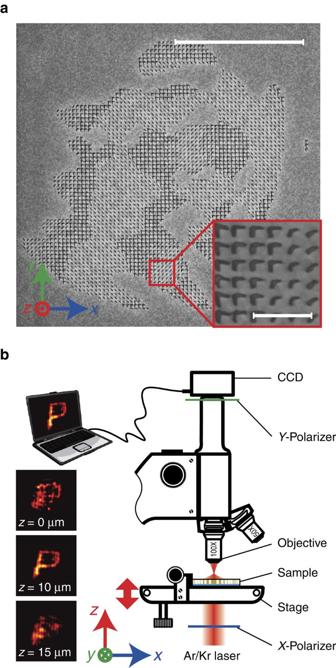Figure 2: Proof-of-concept samples and the experimental set-up. (a) A FE SEM image of a fabricated metasurface for generating a hologram of the letter ‘P’ (scale bar, 5 μm). The inset is a zoomed-in view of the elemental CNAs (scale bar, 500 nm). (b) The schematic of the experimental set-up for viewing the holographic image on the transmission side of the metasurface hologram. The insets on the left are the images at different heights. The upper surface of the sample coincides with thez=0 plane. Figure 2a shows a field-emission scanning electron microscopy (FE SEM) image of the metasurface hologram for generating an image of the letter ‘P’. Note that the metasurface hologram is designed for an operational wavelength of 676 nm, and the thickness of the sample is only about 1/23 the size of the operational wavelength. Figure 2: Proof-of-concept samples and the experimental set-up. ( a ) A FE SEM image of a fabricated metasurface for generating a hologram of the letter ‘P’ (scale bar, 5 μm). The inset is a zoomed-in view of the elemental CNAs (scale bar, 500 nm). ( b ) The schematic of the experimental set-up for viewing the holographic image on the transmission side of the metasurface hologram. The insets on the left are the images at different heights. The upper surface of the sample coincides with the z =0 plane. Full size image Optical characterization of the metasurface hologram The schematic of the measurement system is shown in Fig. 2b and is similar to the set-up used in refs 18 , 35 . The cross-polarized light intensity was measured using a conventional optical microscope with a 100 × objective lens (NA=0.75, WD=0.98 mm) on the transmission side of the sample. The stage resolution along the vertical direction ( z -axis) was 0.5 μm, and the depth of focus for the 100 × objective lens was ~0.5 μm, which is sufficient for our measurements. The sample under test was mounted on the microscope stage with the metasurface side up. The sample was then illuminated from the substrate side with a linearly polarized Ar/Kr laser in continuous-wave mode. Uniform illumination was ensured by using a beam diameter much larger than the size of the metasurface hologram under test. The transmission images from the sample were recorded with a CCD (charge-coupled device) camera. A pair of perpendicular polarizers was placed in the optical path, one before the sample and the second before the CCD camera, to ensure that only the cross-polarized light was collected in the measurement and to eliminate any possible co-polarized background light. Owing to the limited field of view of the microscope, the hologram of each letter was tested individually. By changing the height of the stage in increments of 0.5 μm, we obtained intensity images at different distances from the metasurface on the transmission side. The insets on the left of Fig. 2b are the images obtained at different heights. The light focuses at a height of 10 μm forming a clear image of letter ‘P’ as designed. 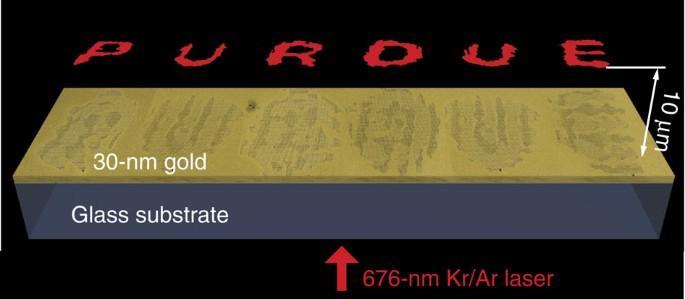Figure 3: Holographic images produced by the experimental metasurface holograms. The image is of the word ‘PURDUE’. The sample is illuminated by a Kr/Ar laser at 676 nm from the glass substrate side. The images are obtained experimentally at a plane 10 μm above the metasurface hologram. The patterns on the gold film are the FE SEM images of the fabricated samples. Figure 3 illustrates the entire sample structure and the holographic images formed above the sample. The patterns on the gold films are the SEM images of the metasurface hologram samples. The images ‘floating’ above the sample are the actual light intensity maps obtained from the optical experiment. 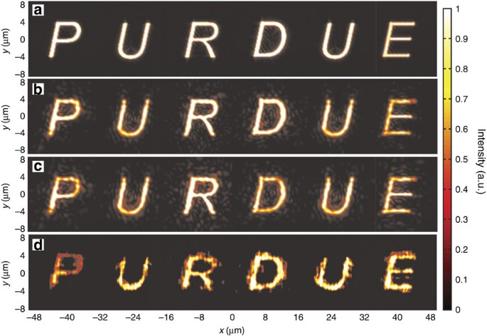Figure 4: Simulated holographic images compared with the experimental images. (a) The simulated holographic images created by an ideal metasurface hologram with smooth phase and amplitude modulations. (b) The simulated holographic images created by a metasurface hologram with an eight-level phase modulation and a four-level amplitude modulation. (c) The simulated holographic images created by a metasurface hologram with an eight-level phase modulation and a two-level amplitude modulation. (d) Holographic images obtained experimentally from the fabricated samples. All the images are taken from the same image plane 10 μm above and parallel to the metasurface hologram. Figure 4a shows the holographic images simulated with an ideal pixelated metasurface hologram using the exact phase and amplitude modulations inside each pixel. In this scenario, the original object is restored almost perfectly. Figure 4b shows the simulated holographic images created by the metasurface hologram using the approximate eight-level phase and four-level amplitude modulations. Figure 4c shows the simulated holographic images created by the metasurface hologram using the approximate eight-level phase and two-level amplitude modulations. Figure 4d depicts the images obtained from our experiments. Although there are two more levels for the amplitude modulation in Fig. 4c compared with Fig. 4b , the quality improvement is limited. The noticeable effect is that the background noise is reduced when more amplitude levels are used, which might be important for more complex holographic images. In our case, two-level amplitude modulation is sufficient for producing clear images. All the images were taken at the same image plane, 10 μm above and parallel to the metasurface hologram. The dimensions of the individual letters obtained from the experiment are <8 × 8 μm 2 , whereas the dimensions of the corresponding metasurface hologram patch for each letter are only about 1.5 times larger (<12 × 12 μm 2 ). The width of the stroke of each letter is ~1 μm. Figure 3: Holographic images produced by the experimental metasurface holograms. The image is of the word ‘PURDUE’. The sample is illuminated by a Kr/Ar laser at 676 nm from the glass substrate side. The images are obtained experimentally at a plane 10 μm above the metasurface hologram. The patterns on the gold film are the FE SEM images of the fabricated samples. Full size image Figure 4: Simulated holographic images compared with the experimental images. ( a ) The simulated holographic images created by an ideal metasurface hologram with smooth phase and amplitude modulations. ( b ) The simulated holographic images created by a metasurface hologram with an eight-level phase modulation and a four-level amplitude modulation. ( c ) The simulated holographic images created by a metasurface hologram with an eight-level phase modulation and a two-level amplitude modulation. ( d ) Holographic images obtained experimentally from the fabricated samples. All the images are taken from the same image plane 10 μm above and parallel to the metasurface hologram. Full size image This proof-of-concept design works at a visible wavelength of 676 nm, and the experimental images match the simulated results. Supplementary Movies 1 and 2 demonstrate the evolution of the images taken at different elevations above the metasurface hologram for both simulated and experimental data. Quantitative analysis An overall efficiency of ~10% (the fraction of the incident energy that contributes into the transmitted holographic image) is achieved in our metasurface hologram design, which is about one order of magnitude greater than the existing metamaterial holograms [9] , [10] . We note that there is no energy going to higher order diffraction (in contrast to the typical hologram implementations). Here, the major issue preventing us from obtaining even higher overall efficiency is the low co-polarization to cross-polarization conversion efficiency of the nanoantennas. A higher overall efficiency is possible through further optimization of the nanoantenna design. We also achieved a signal-to-noise ratio (SNR) of 24.4 in our metasurface hologram sample. The SNR is defined as the ratio of the peak intensity in the image to the standard deviation of the background noise. The background noise was taken from an area of size 60 × 16 μm 2 beside the image. The intensity profile along a cross-section of a stroke, the position of which is indicated in the inset, in letter ‘P’ is shown in Fig. 5 . Understandably, the metasurface hologram with smooth phase and amplitude modulation gives the sharpest feature according to the peak width of the intensity profile. The metasurface holograms with four-level and two-level amplitude modulations have comparable widths of the peaks and both of them are slightly wider peaks than the smooth case. The side lobes are much more significant in the metasurface hologram with two-level amplitude modulation. The experimentally measured intensity profile has a wider peak and more background noise. This is due to fabrication imperfections in the nanoantennas. Nevertheless, it still resolves the stroke quite sharply. 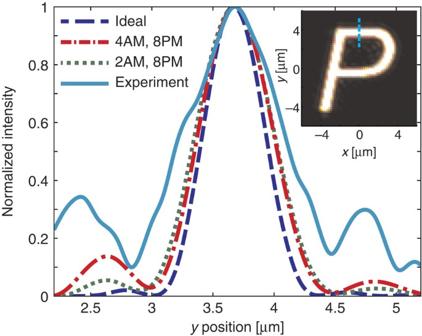Figure 5: Normalized intensity profiles of a cross-section of a stroke in the letter ‘P’. The dashed line is the simulated result from an ideal metasurface hologram with smooth phase and amplitude modulations. The dash-dotted line is the simulated result from a metasurface hologram with an eight-level phase modulation (8PM) and a four-level amplitude modulation (4AM). The dotted line shows the simulated result for a metasurface hologram with an eight-level phase modulation (8PM) and a two-level amplitude modulation (2AM). The solid line is the measured result from the fabricated sample. The dashed line in the inset indicates the position where the cross-section is taken. Figure 5: Normalized intensity profiles of a cross-section of a stroke in the letter ‘P’. The dashed line is the simulated result from an ideal metasurface hologram with smooth phase and amplitude modulations. The dash-dotted line is the simulated result from a metasurface hologram with an eight-level phase modulation (8PM) and a four-level amplitude modulation (4AM). The dotted line shows the simulated result for a metasurface hologram with an eight-level phase modulation (8PM) and a two-level amplitude modulation (2AM). The solid line is the measured result from the fabricated sample. The dashed line in the inset indicates the position where the cross-section is taken. Full size image Our results experimentally prove a viable route for producing complex holograms using nanostructured plasmonic metasurfaces to modulate both amplitude and phase. The proof-of-concept samples built on a CNA design confirm the instrumental features of the proposed method—obtaining high-resolution, low-noise holographic images from ultra-thin, planar nanostructures using subwavelength-scale control of the phase and suppressing the undesired co-polarized light in the cross-polarized images due to the metallic background of the commentary nanoantenna design. It is worth mentioning that a phase-only hologram consisting of plasmonic antennas operating in the near infrared using the weighted Gerchberg–Saxton algorithm has been theoretically studied [36] . Other non-resonant plasmonic structures were also exploited to make conventional binary holograms for generating radially polarized optical beams [37] . Our approach is advantageous in terms of demonstrated flexibility of phase/amplitude control, compactness, SNR, and image resolution. Each nanoantenna in our metasurface hologram only uses an area of 150 × 150 nm 2 , which is the smallest pixel size achieved in these discrete-type holograms. We also note that our metasurface hologram works in both transmission and reflection mode with the same design. Further optimization of our metasurface hologram can pave the way to building even more compact, efficient and versatile optical components for planar optics, conformal nanophotonics and display devices. Design of plasmonic nanoantennas A Babinet-inverted CNA, which is shown schematically in Fig. 6a , has two rectangular arms split at an angle α forming a V shape. The arms have length l and width w . The angle between the symmetry axis of the antenna and the x axis is β . The thickness of the antenna is h . The sharp corners are rounded with fillets of radius w /2 in order to make the design easy to fabricate. Full-wave simulations using the finite element method are performed to obtain accurate designs. The phase shifts as well as the amplitudes of the cross-polarized electric field (normalized to the incident field amplitude) for different α and l with a constant β =45° are plotted as two-dimensional pseudo-colour maps as shown in Fig. 6b,c . From the pseudo-colour maps, we see that the phase shifts and the electric field amplitudes are simultaneously modulated by changing the design parameters (namely α and l ). It is possible to use amplitude modulation with more than two levels by carefully selecting the antenna designs from the parameter space. For example, three sets of designs with different amplitudes are depicted in Fig. 6c as circles, triangles, and squares on the amplitude contour lines. Each set has four antennas which provide relative phase shifts of 0, π /4, π /2, and 3 π /4, respectively (the values of these phase shifts are depicted with a constant offset for ease of reading). The latter four antennas in the unit cell have β =−45°, and the rest of the parameters are the same as those of the first four antennas. They provide relative phase shifts π , 5 π /4, 3 π /2, and 7 π /4, respectively. The designs provide an eight-level phase and four-level amplitude modulation. We note that more phase or amplitude levels can be used if one select denser points in the parameter space, but consequently one need higher resolution in nano-fabrication. In our experiments, for ease of fabrication, we only employed two-level amplitude modulation. The designs we choose for our samples are indicated as circles in Fig. 6c . All the designs we show in this paper have w =30 nm and h =30 nm. 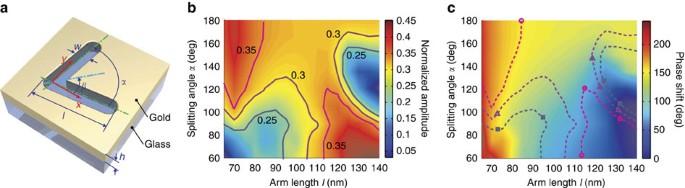Figure 6: Design of Babinet-inverted CNAs. (a) Schematic view of a Babinet-inverted, complementary plasmonic antenna. (b,c) The simulated results for individual antennas on a glass substrate using realistic optical properties for the materials as obtained from experiments. The pseudo-colour maps indicate the amplitudes (b) and the relative phase shifts (c) of the transmitted, cross-polarized electric field due to the change of the arm length of the antennasl(xaxis) and the splitting angleα(yaxis). The solid lines inband the dashed lines incare the amplitude contour lines. The circles, triangles, and squares on the contour lines incindicate the parameters of the antenna designs providing different phases, respectively. The light is incident from the substrate side of the sample and normal to the surface with the electric field polarized in thexdirection. The amplitudes of the cross-polarized electric field are normalized to that of the incident electric field. Figure 6: Design of Babinet-inverted CNAs. ( a ) Schematic view of a Babinet-inverted, complementary plasmonic antenna. ( b , c ) The simulated results for individual antennas on a glass substrate using realistic optical properties for the materials as obtained from experiments. The pseudo-colour maps indicate the amplitudes ( b ) and the relative phase shifts ( c ) of the transmitted, cross-polarized electric field due to the change of the arm length of the antennas l ( x axis) and the splitting angle α ( y axis). The solid lines in b and the dashed lines in c are the amplitude contour lines. The circles, triangles, and squares on the contour lines in c indicate the parameters of the antenna designs providing different phases, respectively. The light is incident from the substrate side of the sample and normal to the surface with the electric field polarized in the x direction. The amplitudes of the cross-polarized electric field are normalized to that of the incident electric field. Full size image Design of the hologram We discretize the virtual object into grids in the image plane, which is 10 μm above the metasurface plane ( z =0 μm) in our case. We regard the virtual object as N point light sources. Each point light source emits linearly polarized, coherent light with a constant phase at a free-space wavelength λ =676 nm. In the three-dimensional space and in the far-field approximation, the electromagnetic field emitted from a point source is proportional to the Green’s function given by , where r s is the position of the point source, r d is a point on the metasurface plane, k =2 π / λ is the wavenumber in the free space. Using the formula above, we can obtain the phase and amplitude of the electric field at the metasurface plane from each light source. The phase, φ ( x , y ,0), and amplitude, E 0 ( x , y ,0), distribution of the total electric field radiated from the virtual object on the metasurface plane is a superposition of electric fields from the N point light sources. We then assign a phase of − φ ( x , y ,0) to each nanoantenna at position ( x , y ) on the metasurface plane. As an example, the required phase and amplitude for the virtual object, letter ‘P’, is depicted in Fig. 2b . How to cite this article: Ni, X. et al. Metasurface holograms for visible light. Nat. Commun. 4:2807 doi: 10.1038/ncomms3807 (2013).